A non-syn-gas catalytic route to methanol production Methanol is an important platform molecule for chemical synthesis and its high energy density also renders it a good candidate as a cleaner transportation fuel. At present, methanol is manufactured from natural gas via the indirect syn-gas route. Here we show that ethylene glycol, a versatile chemical derived from biomass or fossil fuels, can be directly converted to methanol in hydrogen with high selectivity over a Pd/Fe 2 O 3 co-precipitated catalyst. This opens up a possibility for diversification in natural resources for energy-starved countries. The working catalyst contains extremely small 'PdFe' clusters and metal adatoms on defective iron oxide to give the required metal-support interaction for the novel synthesis. The global distribution of natural resources (oil, gas and coal) for energy and chemical provisions is uneven on the biosphere, which has been giving rise to severe political and economic issues in some regions. These non-renewable routes are unlikely to be dominant for a long period of time with an ever increasing world population, reducing natural reserves and prevalent green house gas problems [1] , [2] , [3] , [4] . However, in the meantime before the switch to renewable resources that pose huge scientific and technological challenges, the trend is to manage and diversify these non-renewables for cleaner and more efficient utilizations [4] . Catalytic production of methanol is very important as this high-energy density liquid can be used as a transportation fuel with good volatility (for combustion engines or fuel cells devices), and as a key platform chemical in synthesis [3] . Given the fact that long-term energy security is a key global challenge, the strategic position of methanol is expected to rise [3] . Currently, methanol is synthesized at large scale using natural gas from an energy-inefficient process, which requires an indirect thermal intensive and endothermic step to completely break down the methane to CO/H 2 before they are re-assembled to methanol by the ex-ICI process. From both energetic and resource diversification considerations, it would be ideal to synthesize methanol directly from different carbon-containing resources without any unnecessary atoms reorganization. We are thus interested to explore an alternative non-syn-gas route to utilize ethylene glycol (EG), easily available from biomass or fossil fuels for the methanol production. At present, EG is produced from fossil resources, mainly from an oil-cracking process via ethylene, but can also be made from gas and coal [5] . The gradual depletion of the fossil resources and the emerging environmental concerns have particularly triggered some new developments for its synthesis from biomass as potential renewable process, that is, multi-tonnes scale synthesis from corn carbohydrates as demonstration plants [6] ; from carbohydrates by engineered enzymes [7] ; new synthetic step from cellulose over carbide catalysts [5] , [8] , and so on. Although at present, there is not yet an economic incentive to convert the more costly EG to methanol, the increasing legal and market pulls for methanol utilization may change this position in the future should the science and technology for this step be available. But, the first key technical challenge for this new catalytic process is to identify an active catalytic surface for the efficient C–C cleavage followed by C–H formation to form methanol without further conversion to thermodynamically more stable products such as methane or carbon oxides. Here, we present a unique metal-support interaction of a Pd/Fe 2 O 3 sample prepared by co-precipitation at a controlled pH in aqueous solution. Atomically dispersed Pd in a sol-gel-like matrix formed during the co-precipitation step can be chemically glued with bulk Fe–O–Fe networks. Upon controlled reduction, we show that this material can produce a supported metal phase with extremely high dispersion, ranging from small metal clusters (subnano) down to individual atoms, on a defective iron oxide surface, which has strong metal-support interaction even after heat treatments. As a result, EG can be converted to methanol and ethanol over this catalyst surface. Catalytic studies As seen from Fig. 1a , the conversions of EG molecules in aqueous solution are in general small over all the Pd-containing catalysts under a high pressure of hydrogen, presumably the metal surface is primarily covered with adsorbed hydrogen and water molecules. Various small activities for ethanol production from the hydrogenolysis of EG (C–O bond cleavage followed by C–H formation) were observed over the different samples. Dehydroxylation of one terminal–OH of the diol by oxygen vacancies on oxide support assisted by active hydrogen provided by Pd metal sites in close proximity—is presumably taking place. However, the main product of EG over all the samples is carbon dioxide. It is interesting to note that Pd on iron oxide was the only sample that showed a discernible activity for methanol production (C–C cleavage followed by C–H formation) but with little methane formation. On the other hand, the other samples containing Pd particles on other oxide supports gave no methanol (and only a small quantity of ethanol) but with some degree of methane production. Thus, iron oxide appears to be the essential component for methanol production. We then screened a number of metals supported on iron oxide produced from co-precipitation. As seen from Fig. 1b , the two most promising catalysts Rh/Fe 2 O 3 and Pd/Fe 2 O 3 produced methanol. However, Rh being a metal of stronger adsorptive properties than Pd, according to its d-band centre position [9] , [10] , gave higher conversion but with methane as the primary product. It is noted that metals with stronger intrinsic adsorptive properties are well known to catalyse methane production from hydrocarbons/alcohols with exhaustive hydrogenolysis on their surface [11] . Thus, the combination of Pd and iron oxide clearly shows a good synergetic effect for the production of methanol and ethanol as metastable products, which surprisingly gave even higher selectivity with prolonged testing time in our batch reactor configuration. 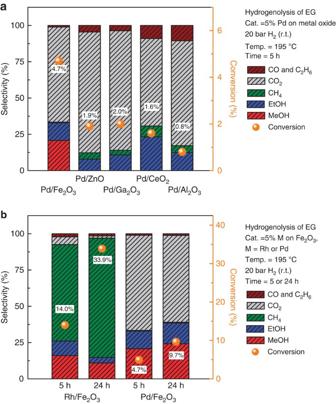Figure 1: Catalytic performances for hydrogenolysis of EG. (a) 5% Pd with different oxides (prepared by co-precipitation); (b) 5% Pd and 5% Rh on iron oxide (prepared by co-precipitation). r.t., room temperature. Figure 1: Catalytic performances for hydrogenolysis of EG. ( a ) 5% Pd with different oxides (prepared by co-precipitation); ( b ) 5% Pd and 5% Rh on iron oxide (prepared by co-precipitation). r.t., room temperature. 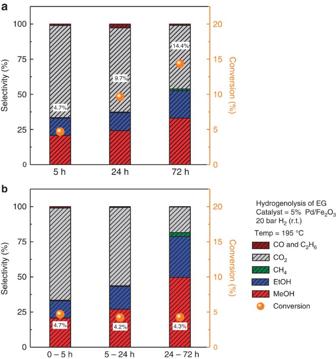Figure 2: Temporal analysis of 5% Pd/Fe2O3in batch-wise hydrogenolysis of EG. (a) Change of gross selectivity over 5% Pd/Fe2O3versus time; (b) time-fraction selectivity over 5% Pd/Fe2O3at different periods. r.t., room temperature. Full size image Figure 2a shows a further improvement in accumulative selectivity of over 50% for the two lower alcohols after the catalyst was tested in a batch reactor for 72 h. Time-fraction analysis in Fig. 2b clearly suggests that the catalyst initially gave higher EG conversions but mainly producing CO 2 . But, between the period of 24 to 72 h, at least 80% selectivity (with methanol selectivity >50%) towards the two lower alcohols at about 4.3% conversion was obtained. The CO 2 produced during the reaction could be owing to the aqueous reforming reaction of EG (C 2 H 6 O 2 +2H 2 O→2CO 2 +5H 2 ) under our reaction conditions [2] , [12] . On the other hand, EG may reduce surface iron oxide in the presence of Pd. Our evidence suggested that the latter reaction has had an important part for the initial production of large quantities of CO 2 . Re-testing the used sample confirmed that the catalyst indeed required an initial long induction period for extensive reduction to reach steady state in order to achieve the good alcohol selectivity ( Supplementary Fig. S1 ); once it was conducted, the catalyst became selective without the need for any further induction. Also, when we pre-reduced our catalyst in hydrogen for a longer duration (72 h) or at a higher temperature, the alcohol selectivity immediately reached the steady state of above 75% with no requirement for the induction. The optimum temperature is around 195 °C, and with repeated testing gives the same alcohol yield. A significant destruction of the products is observed at higher temperature ( Supplementary Fig. S1 ). As far as we are aware, decent conversion of EG or related polyols to the lower alcohols especially to methanol at such high selectivity has not been reported before this work. At present, the methanol/ethanol ratio obtained is above 2:1 and the methanol selectivity can be further optimized. However, for fuel applications there may be no need to separate the two alcohols. The superb catalytic selectivity for this reaction clearly reflects the unusual behaviour of the Pd/Fe 2 O 3 . It is important to investigate the reason(s) for the interesting metal-support interaction observed in yielding methanol at prolonged induction time. Figure 2: Temporal analysis of 5% Pd/Fe 2 O 3 in batch-wise hydrogenolysis of EG. ( a ) Change of gross selectivity over 5% Pd/Fe 2 O 3 versus time; ( b ) time-fraction selectivity over 5% Pd/Fe 2 O 3 at different periods. r.t., room temperature. 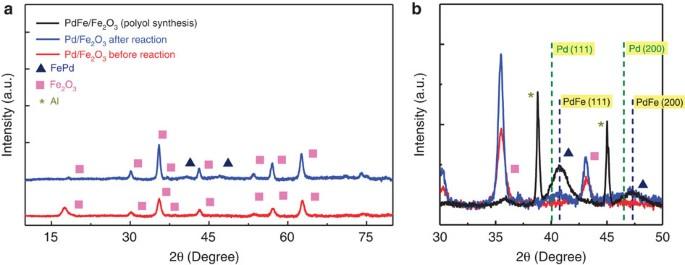Figure 3: XRD spectra of the Pd/Fe2O3. (a) Before and after hydrogenolysis of EG at 195 °C, 20 bar H2(room temperature); (b) enlarged region to show two formed small peaks after reaction corresponding to PdFe rather than Pd; (the high and broad peak at 17° in Pd/Fe2O3before reaction was derived from an air-tight sample holder). Full size image Catalyst characterizations Figure 3a shows an X-ray diffraction (XRD) pattern of the pre-reduced Pd/'Fe 2 O 3 ' (1 h), which gives a 'reduced Fe 2 O 3 ' phase (small Fe 3 O 4 and Fe 2 O 3 phases with air exposure are not easy to be distinguishable hence christened as 'reduced Fe 2 O 3 ') but with no Pd peak observed, indicative of extremely small Pd-containing particles on the reduced iron oxide surface below the detection limit of this technique. On the other hand, two additional broad diffraction peaks marginally differentiable from the background, as shown at 40.76 and 47.09 (see insert), were observed after the sample was tested for this reaction at prolonged time of 72 h (deliberately induced a small degree of sintering). According to the database (JCPDS 88-2335, 65-3253), the diffraction peaks of Pd (1 1 1) and Pd (2 0 0) are at 40.01 and 46.54 (2θ degree) and PdFe (1 1 1) and PdFe (2 0 0) peaks at 40.79 and 47.27 (2θ degree), respectively. Thus, the two peaks matched more closely with those of PdFe than Pd. In addition, XRD peaks of our synthesized PdFe (ca. 4.6 nm) via a polyol process [13] also fitted well with these two peaks. Figure 3: XRD spectra of the Pd/Fe 2 O 3 . ( a ) Before and after hydrogenolysis of EG at 195 °C, 20 bar H 2 (room temperature); ( b ) enlarged region to show two formed small peaks after reaction corresponding to PdFe rather than Pd; (the high and broad peak at 17° in Pd/Fe 2 O 3 before reaction was derived from an air-tight sample holder). Full size image It is thus evident that there must be a deep reduction of Pd/Fe 2 O 3 by EG (itself oxidized to CO 2 ) assisted by Pd to give PdFe nanoparticles during the induction period, which accounts for the poor initial alcohol selectivity. It is noticed that extensive reduction of pure Fe 2 O 3 by hydrogen should not take place under our pre-reduction or testing conditions [14] . Hydrogen temperature-programmed reduction (TPR) in Fig. 4a indeed shows no reduction of Fe 2 O 3 until the temperature is about 340 °C. It is interesting to note that the presence of Pd appears to catalyse the reduction of Fe 2 O 3 more readily. The reduction temperature was shifted to around 130 °C owing to the incorporation of Pd. This implies that a catalysed reduction of some Fe 3+ to primarily Fe 2+ to form the 'Fe 3 O 4 ' phase but also to Fe o associated with Pd o to produce PdFe in hydrogen under our pre-reduction/testing conditions. 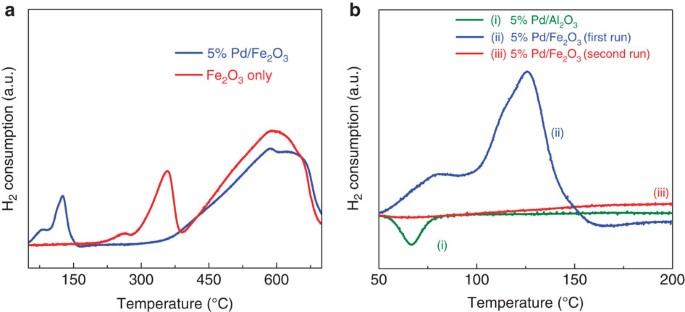Figure 4: TPR measurements. (a) H2-TPR profiles of Fe2O3and Pd/'Fe2O3; (b) first and second repeated TPR profiles of Pd/'Fe2O3' in H2after the temperature-programmed heating terminated at 200 °C as compared with TPR profiles of Pd/Al2O3. Figure 4b clearly shows the absence of typical hydrogen evolution peak of β-Pd hydride [15] (pure Pd particles should readily take up hydrogen to form hydride at room temperature) as compared with alumina-supported Pd at around 70 °C (negative peak) in the second TPR profile of the same Pd/'Fe 2 O 3 ' sample without exposure to air, the fact is again consistent with the formation of highly-dispersive PdFe clusters in the sample. Figure 4: TPR measurements. ( a ) H 2 -TPR profiles of Fe 2 O 3 and Pd/'Fe 2 O 3 ; ( b ) first and second repeated TPR profiles of Pd/'Fe 2 O 3 ' in H 2 after the temperature-programmed heating terminated at 200 °C as compared with TPR profiles of Pd/Al 2 O 3 . Full size image We have carried out extended X-ray absorption fine structure (EXAFS) characterization at the Pd K-edge (24,350 eV) on our samples before (poor methanol selectivity) and after extensive reduction (good methanol selectivity) as compared with a commercial 5% Pd/C catalyst. We were particularly interested to estimate the size of Pd-containing particles based on the analysis of coordination number (CN) derived from EXAFS data, which should be more representative than those from the transmission electron microscopy (TEM) (regional analysis) and XRD (small size escapes from detection). Based on the refined parameters included in Table 1 , it is noted that the commercial Pd/C with 2-nm Pd particles gives the CN of ca. 8.0 at Pd–Pd distance of 2.73 Å from the first shell analysis. The results are consistent with the detailed size estimations of supported Pd particles from a recent EXAFS study alongside with other multiple techniques including gas adsorption, TEM and XRD [16] . Similarly, the derived CN of ca. 3.5 reflects the four-fold symmetry (square planar) of –PdO 4 – in our non-reduced gel form. It is very interesting to observe an extremely low average CN of Pd–Pd distance in the sample after the pre-reduction within the acceptable R- and D-W factors. According to their model (cubooctahedral shape of Pd was assumed) and calibration curve, such small CN corresponds to Pd particles smaller than ca. 1 nm, hence they are in metallic cluster regime (or groups of adatoms). Perhaps, the other most striking features we observed are the direct observation for a Pd–Fe distance (CN=1.0) at 2.59 Å and a shorter, distorted Pd–Pd distance (CN=1.9) at 2.66 Å after reduction, confirming the formation of 'PdFe' clusters. In addition, our CO chemisorption measurements on the sample after extensive reduction at 200 °C (82.61 μmol g −1 cat.) clearly reflect the attenuation in the CO uptake value as compared with the same sample with the reduction at 40 °C (135.33 μmol g −1 cat. with only the formation of Pd 0 ). This matches with the same observation of the literature describing the dilution and electronic effects of Pd and Fe atoms to CO molecules on 'PdFe' surface [17] . It should be noted that such small 'PdFe'-containing clusters on oxide surface could be very different from those thermodynamic stable PdFe alloy with defined structures, stoichiometries and morphologies. Table 1 EXAFS analyses for Pd K-edge. Full size table High-angle annular dark field scanning TEM was used to acquire the detailed microscopic view and morphology of the Pd/'Fe 2 O 3 ' catalyst particles after pre-reduction. Using this imaging technique, a JEOL JEM-2200MCO aberration-corrected transmission electron microscope indeed revealed a large number of small metal particles in the observable thin areas of 'Fe 2 O 3 '. The metal particles ranged in size from ca. 0.5 to 2.5 nm in diameter, with particles of 0.5–1.5 nm being the most commonly measured size, as shown in Supplementary Fig. S2 . Energy-dispersive X-ray spectroscopy confirms that the particles consist predominantly of Pd and Fe, although any Fe content could not be unambiguously determined owing to the underlying iron oxide support. The direct visualization of extremely small metal clusters (groups of atoms) and occasionally even single atoms around the edges of the clusters on the reduced 'Fe 2 O 3 ' surface under higher magnification could be made. This result matched with the observation of the low CN derived from the EXAFS data. 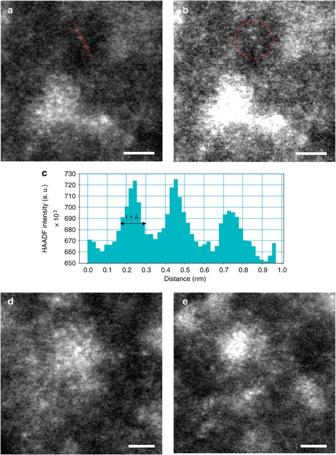Figure 5: HAADF–STEM imaging of Pd/'Fe2O3' catalyst. (a) Typical area of the specimen containing irregular atomic clusters with three distinctive surface adatoms; (b) the same raw data as (a) with the image contrast enhanced to visualize the three single adatoms. The circle highlights the three single adatoms on the 'Fe2O3' surface; (c) line profile along the line marked in (a), showing the three distinct isolated atoms, each with a half peak width of 1.1 Å; (d) and (e) represent typical irregular groups of atoms as clusters found in the catalyst material. Scale bar, 1 nm. Figure 5a shows typical small particles of Pd around 1–2 nm in size; the structure and shape of the particles are very irregular and individual atoms around the particle perimeter can be seen. In Fig. 5b , the image contrast level has been increased to aid the identification of small clusters of metal atoms on the surface, such as those highlighted within the marked circle. An intensity line profile as marked in Fig. 5a is plotted in Fig. 5c and suggests a group of three isolated adatoms, each with a reproducible half peak width of 1.1±0.1 Å. However, it was unable to ascertain whether Pd or Fe or mixed adatoms were produced based only on this microscopic study. The contrast level relative to the support and that of single adatoms suggests that the particle consists generally of one or two layers of metal atoms as clusters. Figure 5d,e shows further representative areas of the catalyst again with an unusually high density of ultra-small metal clusters composed of atom groups on the surface Pd/'Fe 2 O 3 '. Zhang and co-workers have recently reported dispersed single Pt atoms on iron oxide using a similar preparative method as ours and they attributed the observed high activity for CO oxidation to the catalysis by these single metal sites [18] . Although we cannot discount the single metal site catalysis of this hydrogenolysis, more complex steric requirements for adsorption and catalysis of this substrate with metal sites are expected [19] . It is also noted that there is no literature reported for homogeneous single metal site catalysts to activate EG to methanol in hydrogen. In addition, the need for extensive pre-reduction time (long activation time) and the formation of corresponding high-density PdFe clusters on surface before the detection of methanol support the fact that the PdFe clusters are the active species responsible for methanol production. Figure 5: HAADF–STEM imaging of Pd/'Fe 2 O 3 ' catalyst. ( a ) Typical area of the specimen containing irregular atomic clusters with three distinctive surface adatoms; ( b ) the same raw data as ( a ) with the image contrast enhanced to visualize the three single adatoms. The circle highlights the three single adatoms on the 'Fe 2 O 3 ' surface; ( c ) line profile along the line marked in ( a ), showing the three distinct isolated atoms, each with a half peak width of 1.1 Å; ( d ) and ( e ) represent typical irregular groups of atoms as clusters found in the catalyst material. Scale bar, 1 nm. Full size image In order to obtain a correlation on the quantity of methanol production with the amount of PdFe clusters made on the catalyst surface, samples tested for the EG hydrogenolysis at different durations (with different methanol selectivities) were then carefully quenched and analysed by XPS. 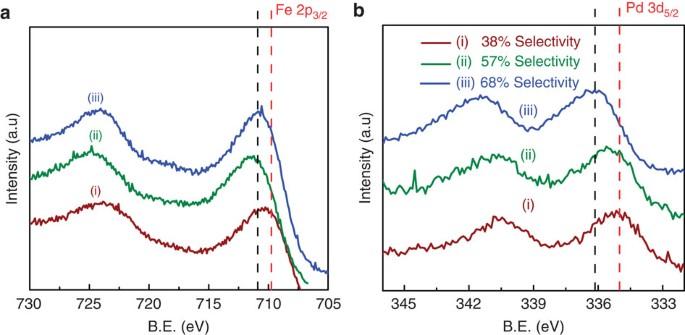Figure 6: XPS spectra of Pd/Fe2O3catalyst at different hydrogen pre-reduction times (1, 5 and 48 h). The spectra are evaluated at 195 °C for 24 h (corresponding with different alcohols selectivities). All spectra were calibrated to adventurous C 1-s peak at 284.5 eV with the application of electron shower gun to reduce charging effect of the samples. (a) Fe 2p3/2region. The red dash line corresponds to the binding energy of Fe 2p3/2and the dark dash line corresponds to Fe 2p3/2in PdFe alloy from the literature (NIST database) values20; (b) Pd 3d5/2region. The red dash line corresponds to the binding energy of Pd 3d5/2and the dark dash line corresponds to Pd 3d5/2in PdFe alloy from the literature (NIST database) values20. Figure 6 indicates that the binding energies of Pd and Fe are both shifted to higher values according to literature values, indicative of 'PdFe' alloy-like formation [20] , [21] , [22] , [23] . There was unfortunately no clear correlation on the shift of binding energy of Fe 2p 3/2 ( Fig. 6a ) with respect to the methanol selectivity owing to the interference from bulk iron oxide background. On the other hand, the progressive binding energy shift of Pd 3d 5/2 of 335.16 eV (pure Pd) to the converging value of 336.17 eV shown in Fig. 6b (matched with those value of PdFe sample ( ca. 4.6 nm) and extensively hydrogen pre-reduced sample) clearly suggested that the increasing amount of PdFe [21] on surface corresponded well with the raising methanol selectivity. Figure 6: XPS spectra of Pd/Fe 2 O 3 catalyst at different hydrogen pre-reduction times (1, 5 and 48 h). The spectra are evaluated at 195 °C for 24 h (corresponding with different alcohols selectivities). All spectra were calibrated to adventurous C 1-s peak at 284.5 eV with the application of electron shower gun to reduce charging effect of the samples. ( a ) Fe 2p 3/2 region. The red dash line corresponds to the binding energy of Fe 2p 3/2 and the dark dash line corresponds to Fe 2p 3/2 in PdFe alloy from the literature (NIST database) values [20] ; ( b ) Pd 3d 5/2 region. The red dash line corresponds to the binding energy of Pd 3d 5/2 and the dark dash line corresponds to Pd 3d 5/2 in PdFe alloy from the literature (NIST database) values [20] . Full size image It is thus clearly demonstrated from this work that methanol can be synthesized with high selectivity and a decent conversion by the direct hydrogenolysis of biomass-derived EG over Pd/Fe 2 O 3 , opening up a new diversity for activation of other carbon-containing resources (biomass and oil) from natural gas using the syn-gas route. From a mechanistic viewpoint, conversion of an EG molecule to methanol or ethanol requires C–C or C–O bond breakage with C–H formation over the catalytically active site(s) on Pd/'Fe 2 O 3 ' in a highly cooperative and concerted manner, otherwise the extensive surface adsorption and degradation of the substrate and intermediates on large metal catalyst surfaces will lead to the more thermodynamically stable CO 2 or CH 4 formation [19] . The importance is to eliminate or substantially reduce the formation of the stable products by the use of extremely well-dispersed Pd-containing clusters/atoms. We observe that a Pd/Fe 2 O 3 catalyst prepared by simple co-precipitation displays an unusual material interaction, long described as 'strong metal-support interaction'. Our evidence suggests the formation of extremely dispersed PdFe clusters and adatoms on iron oxide surface during catalysis. Their presence undoubtedly indicates a degree of chemical species exchange and reconstruction at the interface between the metal and oxide support, giving a kind of 'chemical definition' of this metal-support interaction. The observed atomic levels of dispersion on iron oxide are surprising given the fact that the sample had experienced various heat pre-treatments. It is believed that a sol-gel-like chemistry through hydrolysis and cross condensation during the co-precipitation of iron and palladium nitrates has a crucial role in the dispersion [24] , as shown in Supplementary Fig. S6 . The formation of small but catalytically active PdFe clusters at high surface concentration can offer enhanced activity/selectivity owing to electronic modification of Pd-band-like structure [9] , [25] . The thermal refractory nature of the alloy clusters can also reduce their surface mobility under our moderate testing conditions otherwise large particles would have been obtained. The formation of these small PdFe clusters or subnanoparticles is expected to be extremely important for the methanol production in the new synthetic step. The recent Density Functional Theory (DFT) calculations clearly suggest the kinetic adsorption of C–O bonds of EG is much favourable than both C–H and C–C adsorptions over extended (111) metal surfaces [19] . The bidentate nature of adsorbed EG forces the C–O bonds into an angle more perpendicular to the plane of the surface than one C–O bond in the case of monoalcohols on a flat metal surface. This facilitates activation of C–O bonds but destabilizes the approach of α H in C–H or α C in C–C at the other end of the molecule to the terrace metal sites, giving the undesirable cleavages. On the other hand, the relaxation of the steric constraints on small cluster/subnano metal would therefore facilitate C–C activation, leading to scissoring of the molecule followed by C–H formation to methanol on their low coordination sites. In addition, surface oxygen vacancies are expected to be formed simultaneously with the Fe 3+ reduction in close vicinity to the formed PdFe clusters from the support surface (refer to the TPR) owing to the maintenance of electrical neutrality, which will assist adsorption of EG molecules [26] . As EG is the simplest representative of biomass-derived polyols, selective cleavage of C–C in other biomass molecules to form methanol over the small surface PdFe clusters could be achieved. In light of this work, it would be interesting to elucidate the recent reported 'special metal-support interactions' of Au and Ag clusters on a wide range of exciting catalysis in literature [27] , [28] . In conclusion, we report a new catalytic methanol production process over Pd/Fe 2 O 3 with a strong and unique metal-support interaction. Further studies are warranted to optimize productivity for methanol and evaluate catalyst stability under industrial applicable conditions but this novel catalytic capability may open up a new way to convert other carbon-containing natural resources to methanol apart from the established natural gas process via the syn-gas route. As a result, oil/coal-based EG and especially the biomass-based EG with stronger environmental incentives can be used to produce this strategic important fuel or chemical. In addition, the combined selectivity to methanol/ethanol of 80% with the rest of CO 2 and H 2 co-products from aqueous reforming may also allow reduction or elimination of the need for expensive hydrogen gas input (hydrogen is balanced for this product distribution), rendering the catalytic process promising at this stage. Synthesis of metal oxide-supported catalysts made by co-precipitation Typical synthesis for 1 g of 5% Pd/Fe 2 O 3 catalyst was carried out as follows: 0.3309 g of Pd(NO 3 ) 2 solution from Alfa Aesar (15.11wt% Pd) and 5.071 g of Fe(NO 3 ) 3 .9H 2 O from Sigma Aldrich were dissolved in a 200 ml deionized water at room temperature under stirring. Then, 1.0 M Na 2 CO 3 solution was added dropwise to the mixed solution until the pH of the final solution reached ca . 9.0. After stirring and aging for overnight at room temperature, the resulting precipitate (denoted as Pd/Fe(OH) x ) [29] was filtered, washed with 200 ml deionized water each for ten times, air-dried at 110 °C overnight, gently grounded by pestle and mortar, and calcined in air at 300 °C for 2 h. The dried calcined powder (Pd/Fe 2 O 3 ) was then pre-reduced in a flowing stream of 33% H 2 /N 2 at a steady rate of 60 ml min −1 in a tube furnace at 200 °C for 1, 5, 48 or 72 h, respectively. The furnace was then cooled down to room temperature and the powder was transferred into a glove box for storage before the catalytic testing. The as-reduced catalyst was denoted as Pd/'Fe 2 O 3 '. Handling of pre-reduced Pd/'Fe 2 O 3 ' samples Our early experiments suggested that the pre-reduction treatments (temperature and duration) are extremely important, which affect initial catalytic activity of the samples (induction time). As a result, all samples after pre-reduction were then handled and transferred with extreme care without contacting air. For example, the transfers of the samples for XPS, TEM, XRD and EXAFS studies were conducted in an inert gas using a glove bag and/or air-tight sample holders (XRD and EXAFS) before their analyses. Catalytic testing for hydrogenolysis of EG The hydrogenolysis reaction was carried out in liquid phase using a 160 ml autoclave high-pressure reactor fitted with glass liner. In a typical experiment, 30 ml of EG solution (0.85 mol l −1 ) and 0.50 g of catalyst were loaded in a glove box. The reactor was flushed with pure hydrogen to remove any traces of oxygen. The autoclave was pressurized to 20 bars of hydrogen at room temperature. Then, it was heated up to 195 °C and allowed to react for 24 h with a constant stirring. Products analysis After reaction, the autoclave was cooled down to −60 °C by dry ice/acetone bath. Here, the gas phase was analysed by a Perkin Elmer Autosystem XL Arnel Gas phase GC-FID-Methanator in order to determinate the concentrations of CO, CH 4 and CO 2 after the reaction. The liquid phase was analysed by a Perkin Elmer 200 series HPLC equipped with a refractive index detector where a 0.60 ml of 58 mmol l −1 sucrose solution was added as an external standard to determinate the concentration of EG, methanol and ethanol after the reaction. The mass balance of this typical catalytic batch reaction of over 95% was ensured. Powder XRD analysis The powder sample was placed in an air-tight sample holder prepared in a glove box. XRD data were then collected using a PANalytical X'Pert Pro diffractometer, operating in Bragg–Brentano focusing geometry and using Cu Kα radiation ( λ =1.5418 Å) from a generator operating at 40 kV and 40 mA. EXAFS analysis EXAFS measurement at the Pd K-edge (24530 eV) were performed on B18 beamline at Diamond Light Source (Diamond, UK) to obtain information about the local structure of Pd catalysts (the nearest-neighbour interatomic distances and CN), which was then used to estimate the size of Pd particles. The Diamond installation comprises a 3 GeV electron storage ring with typical currents of 200 mA. The B18 is a bending magnet beamline that has been designed to deliver monochromatic X-rays in the energy range of 2 to 35 keV. A Si (311) double-crystal monochromator was used for energy selection with the resolution of 1 eV. X-ray absorption spectroscopy data were collected at the Pd K-edge at ambient temperature in transmission mode using optimized ionization chambers as detectors. Fluorescence spectra were acquired using I0 and a high-count rate fluorescence 9-element Ge detector windowed on the Pd K-edge fluorescence peaks. Acquisition time of the XAS spectrum for each sample was about 40 min, 8–12 scans were collected for each sample. The EXAFS data analysis was performed using IFEFFIT 1 with Horae packages 2 (Athena and Artemes) [30] , [31] . All spectra were calibrated with Pd foil as the reference to avoid small energy shifts of the nano catalyst. The amplitude parameter was obtained from EXAFS data analysis of Pd foil (with known CNs that were fixed during analysis) to be 0.84, which was used as a fixed input parameter in all fits to allow CN refinement. The k 3 -weighted spectra were Fourier transformed within the limits 2< k <15 and 1< R <3. In this work, we perform only a first shell data analysis under the assumption of single scattering. For the curve-fitting analysis, the empirical phase shift and amplitude functions for Pd–Fe bond and Pd–Pd bond were extracted from the data for PdFe alloy and Pd foil, respectively. Errors in the analysis were estimated by R factor. How to cite this article: Wu, C.-T. et al . A non-syn-gas catalytic route to methanol production. Nat. Commun. 3:1050 doi: 10.1038/ncomms2053 (2012).